High doses of CpG oligodeoxynucleotides stimulate a tolerogenic TLR9–TRIF pathway CpG-rich oligodeoxynucleotides activate the immune system, leading to innate and acquired immune responses. The immune-stimulatory effects of CpG-rich oligodeoxynucleotides are being exploited as a therapeutic approach. Here we show that at high doses, CpG-rich oligodeoxynucleotides promote an opposite, tolerogenic response in mouse plasmacytoid dendritic cells in vivo and in a human in vitro model. Unveiling a previously undescribed role for TRIF and TRAF6 proteins in Toll-like receptor 9 (TLR9) signalling, we demonstrate that physical association of TLR9, TRIF and TRAF6 leads to activation of noncanonical NF-κB signalling and the induction of IRF3- and TGF-β-dependent immune-suppressive tryptophan catabolism. In vivo , the TLR9–TRIF circuit—but not MyD88 signalling—was required for CpG protection against allergic inflammation. Our findings may be relevant to an increased understanding of the complexity of Toll-like receptor signalling and optimal exploitation of CpG-rich oligodeoxynucleotides as immune modulators. Toll-like receptors (TLRs) are part of the innate immune system, and they belong to the pattern recognition receptor family. This family recognizes and binds conserved pathogen-associated molecular patterns, which are not generated by the host, and are restricted and essential to microorganisms. TLR9, which recognizes unmethylated cytosine–phosphate–guanosine (CpG) motifs, is a very promising target for therapeutic activation. Stimulation of TLR9 activates human plasmacytoid dendritic cells (pDCs) and B cells, and results in potent Th1-type immune reactivity and antitumor responses in mouse tumour models and in patients [1] . While CpG-rich oligodeoxynucleotides (CpG-ODNs) are potent immune activators in mice—accelerating and boosting antigen-specific immune responses by 5–500-fold [2] —their stimulatory effects are often less dramatic in humans, and this disparity between rodents and mammals has been attributed to differences in TLR9 expression in the different species [3] . Immunotherapeutic applications of CpG-ODN TLR9 agonists include not only approaches to enhance immune responses but also immunosuppressive strategies for treating allergy [4] and autoimmunity [5] . In both mice and humans, the immunosuppressive activity of TLR9 agonists has been attributed to the regulatory function of indoleamine 2,3-dioxygenase 1 (IDO1) [6] , [7] , which is reportedly activated by CpG mainly as a function of its route of administration, with systemic application strongly suppressing—rather than enhancing—T-cell immunity [7] , [8] . Human pDCs stimulated with TLR7 or TLR9 ligands induce CD8 + LAG-3 + Foxp3 + CTLA-4 + regulatory (Treg) cells that suppress alloreactive memory T cells via an IDO1-dependent mechanism [9] . Unlike TLR9, TLR7 is targeted by synthetic GpC-ODNs, yet its univocally tolerogenic signalling exploits IDO1 as a downstream effector mechanism [10] . In the present study, by using purified mouse pDCs treated with CpG in vitro , we demonstrate a clear-cut dichotomy of pDC-based immunotherapy in vivo —immunostimulation as opposed to IDO1-dependent immunosuppression—depending on ODN dosages. This could be traced to the respective dominance of interleukin (IL)-23 versus transforming growth factor (TGF)-β production. Differential cytokine production was, in turn, underlain by disparate modalities of MyD88- versus TRIF-dependent signal transduction, resulting in mutually antagonistic pathways of canonical and noncanonical NF-κB activation in the pDCs. Different doses of CpG promote opposite effects At least three structurally distinct classes of CpG-ODNs have been described in primates. ‘B’ type ODNs encode multiple CpG motifs on a phosphorothioate backbone, which replaces and stabilizes the phosphodiester backbone present in naturally occurring A-type CpG-ODNs. B-type CpG-ODNs activate pDCs and trigger B cells to proliferate and secrete cytokines [2] . Preliminary evidence indicated that splenic pDCs (CD11c + mPDCA-1 + 120G8 + ) are made immunogenic by overnight exposure to 1 μg ml −1 —but not 10 μg ml −1 —of B-type CpG-ODN 1826 in a model system of skin test reactivity to the tumour and self P815AB nonapeptide [11] , [12] , such that peptide-pulsed pDCs would effectively sensitize recipient hosts to intrafootpad challenge with the peptide in saline ( Supplementary Fig. S1 ). As high-dosage CpG-ODN 1826 manifests pDC-dependent therapeutic activity in experimental autoimmunity [13] , we examined whether the higher concentration, 10 μg ml −1 , of CpG-ODN would, in fact, confer tolerogenic activity on the pDCs. Cells were treated with 1 or 10 μg ml −1 CpG-ODN, and admixed with spontaneously tolerogenic CD8 + DCs ( Fig. 1a ) or immunogenic CD8 − DCs ( Fig. 1b ) in a skin test assay. The immunoadjuvant effect selectively conferred on pDCs by 1 μg ml −1 of CpG-ODN was strong enough to make cells surmount suppression by the CD8 + DC fraction. In contrast, the higher CpG dosage induced such strong suppressive effects on the pDCs that immunogenic peptide presentation by coadministered CD8 − DCs could no longer be observed. The suppressive potential conferred by CpG-ODN on pDCs was contingent on functional IDO1, as the effect was ablated by treating the CpG-conditioned pDCs with Ido1 -specific small-interfering (si)RNA or by the IDO1 inhibitor 1-methyl-tryptophan ( Fig. 1b ; Supplementary Fig. S2 ). Both the lower-dose immunostimulant activity ( Supplementary Fig. S3a ) and the higher–dose–suppressive effect ( Supplementary Fig. S3b ) of CpG-ODN 1826 were shared by the corresponding ODN on a phosphodiester backbone (CpG-A). Two non-CpG-ODNs, namely a negative control ODN (nc-ODN; a scrambled sequence from ODN 1826) and a GpC-ODN (in which the CpG motif had been replaced by GpC), both on a phosphorothioate backbone, lacked stimulatory activity ( Supplementary Fig. S4 ). As expected [10] , the GpC-ODN manifested IDO1-dependent tolerogenic activity in a dose-independent fashion (that is, at both 1 and 10 μg ml −1 ) ( Fig. 1c ). Importantly, the nc-ODN lacked suppressive activity and, overall, showed no activity at all in our model system ( Fig. 1c ). The dual activity of CpG-ODN in our setting could be mimicked by lipopolysaccharide-free, bacterial DNA, which likely represents the physiological TLR9 ligand ( Supplementary Fig. S5 ). This confirmed the duality of function in splenic pDCs treated with CpG-ODN and the IDO1 dependency of the tolerogenic effect. 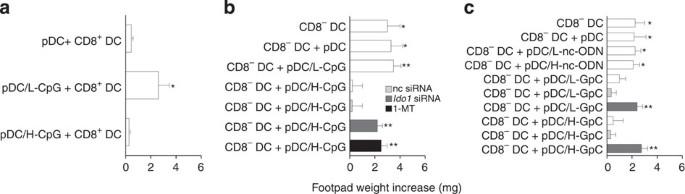Figure 1: Dual activity of pDCs treated with respective low or high doses of CpG 1826in vitro. Splenic CD11c+DCs from DBA/2 mice were fractionated according to mPDCA-1 or CD8 expression, pulsed with the P815AB peptide and transferred intravenously into recipient hosts to be assayed at 2 weeks for footpad reactivity to soluble peptide challenge. (a) Transferred pDCs cells were either untreated or treated overnight with 1 (pDC/L-CpG) or 10 (pDC/H-CpG) μg ml−1of ODN and were used in combination with a minority fraction (5%) of tolerogenic CD8+DCs. (b) According to a similar design, after overnight exposure to 1 or 10 μg ml−1CpG, the pDCs were assayed for suppressive activity of immunogenic peptide presentation by the CD8−DC fraction. In this setting, the suppressive potential conferred on pDCs by 10 μg ml−1CpG was ablated by silencingIdo1expression or by pDC treatment with the competitive IDO inhibitor 1-methyl-tryptophan (1-MT). (c) The modified, non-CpG ODN 1826 (GpC ODN), but not the scrambled, nc sequence of the 1826 oligo (nc-ODN), displays dose-independent suppressive activity contingent on functional IDO1. The experimental design is the same as that in (b). The asterisks (*P<0.01 and **P<0.001; experimental versus control footpads; two-tailed pairedt-test) indicate the occurrence of a positive skin test reaction as a result of unopposed presentation of the peptide by the pDCs made immunogenic by CpG or by the spontaneously immunogenic CD8−DC fraction. Data are mean values±s.d. of three experiments. Figure 1: Dual activity of pDCs treated with respective low or high doses of CpG 1826 in vitro . Splenic CD11c + DCs from DBA/2 mice were fractionated according to mPDCA-1 or CD8 expression, pulsed with the P815AB peptide and transferred intravenously into recipient hosts to be assayed at 2 weeks for footpad reactivity to soluble peptide challenge. ( a ) Transferred pDCs cells were either untreated or treated overnight with 1 (pDC/L-CpG) or 10 (pDC/H-CpG) μg ml −1 of ODN and were used in combination with a minority fraction (5%) of tolerogenic CD8 + DCs. ( b ) According to a similar design, after overnight exposure to 1 or 10 μg ml −1 CpG, the pDCs were assayed for suppressive activity of immunogenic peptide presentation by the CD8 − DC fraction. In this setting, the suppressive potential conferred on pDCs by 10 μg ml −1 CpG was ablated by silencing Ido1 expression or by pDC treatment with the competitive IDO inhibitor 1-methyl-tryptophan (1-MT). ( c ) The modified, non-CpG ODN 1826 (GpC ODN), but not the scrambled, nc sequence of the 1826 oligo (nc-ODN), displays dose-independent suppressive activity contingent on functional IDO1. The experimental design is the same as that in ( b ). The asterisks (* P <0.01 and ** P <0.001; experimental versus control footpads; two-tailed paired t -test) indicate the occurrence of a positive skin test reaction as a result of unopposed presentation of the peptide by the pDCs made immunogenic by CpG or by the spontaneously immunogenic CD8 − DC fraction. Data are mean values±s.d. of three experiments. Full size image IL-23 and TGF-β dependency of opposing activities of CpG Flexibility in DC presentation programs mostly reflects autocrine effects by a set of cytokines, which either reinforce or subvert a default presentation profile [14] . Typically, the IL-12–IL-23 pair [15] and IL-6 [16] induce immunogenic presentation, whereas TGF-β [17] and type I or type II interferons (IFNs) [18] promote tolerance, via transcriptional [19] or posttranslational [20] regulation of IDO1. After pDC exposure to CpG-ODN, GpC-ODN or nc-ODN, at 1 or 10 μg ml −1 , transcripts specific for IL-6, IL-10, IL-23 p19, IFN-α, IFN-β, IFN-γ and TGF-β were measured by real-time PCR ( Fig. 2a ). Cytokine content in 24-h culture supernatants was measured by enzyme-linked immunosorbent assay (ELISA) ( Fig. 2b ). At the transcriptional level, low-dose CpG was found to promote Il23a induction, whereas high-dose CpG induced Tgfb1 . However, while secreted IL-23 could be found in the early culture supernatants, TGF-β would apparently occur in a large latent complex or as a biologically active cell surface molecule [21] , as demonstrated by concomitant staining for the intracellular cytokine ( Fig. 2c and Supplementary Fig. S6 ). However, in 72-h culture supernatants, we could document CpG-induced TGF-β activity in a specific in vitro assay ( Fig. 2d ). On the other hand, pDCs stimulation by GpC resulted in measurable TGF-β in culture supernatants at as early as 24 h, further underlining the qualitatively different mechanism of action of CpG and GpC in TLR signalling [10] . 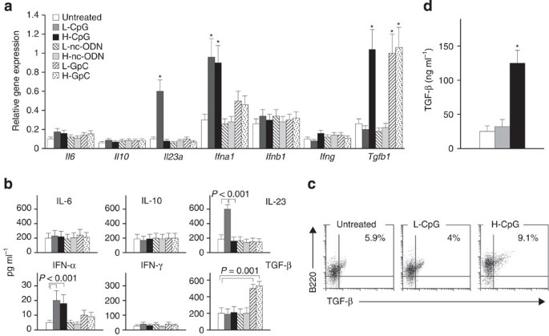Figure 2: Cytokine expression profiles of pDCs treated with low or high doses of CpG or GpC. (a)Il6,Il10,Il23a,Ifna1,Ifnb1,IfngandTgfb1transcripts were evaluated in pDCs treated with 1 or 10 μg ml−1of CpG, nc-ODN or GpC for 6 h. IL-6, IL-10, IL-23 p19, IFN-α, IFN-β, IFN-γ and TGF-β mRNAs were quantified by real-time PCR usingGapdhnormalization. Data (means±s.d. from four experiments) are presented as transcriptional expression of the different cytokines relative to basal cytokine transcript amount in unstimulated cells. *P<0.005; Student’st-test. (b) pDCs were assayed for cytokine release after CpG, nc-ODN or GpC exposure. Data are means±s.d. from four experiments. (c) Intracellular TGF-β staining profiles of B220+pDCs treated with 1 or 10 μg ml−1of CpG for 24 h. Shown in upper right quadrants are percentages of double-positive cells. One experiment is shown representative of six, all of which are visualized by scatter plot inSupplementary Fig. S6. (d) Production of TGF-β by pDCs untreated or treated with 1 (pDC/L-CpG) or 10 (pDC/H-CpG) μg ml−1of ODN. Supernatants were harvested at 72 h after stimulation and assayed for active TGF-β. *P<0.01; Student’st-test. Figure 2: Cytokine expression profiles of pDCs treated with low or high doses of CpG or GpC. ( a ) Il6 , Il10 , Il23a , Ifna1 , Ifnb1 , Ifng and Tgfb1 transcripts were evaluated in pDCs treated with 1 or 10 μg ml −1 of CpG, nc-ODN or GpC for 6 h. IL-6, IL-10, IL-23 p19, IFN-α, IFN-β, IFN-γ and TGF-β mRNAs were quantified by real-time PCR using Gapdh normalization. Data (means±s.d. from four experiments) are presented as transcriptional expression of the different cytokines relative to basal cytokine transcript amount in unstimulated cells. * P <0.005; Student’s t -test. ( b ) pDCs were assayed for cytokine release after CpG, nc-ODN or GpC exposure. Data are means±s.d. from four experiments. ( c ) Intracellular TGF-β staining profiles of B220 + pDCs treated with 1 or 10 μg ml −1 of CpG for 24 h. Shown in upper right quadrants are percentages of double-positive cells. One experiment is shown representative of six, all of which are visualized by scatter plot in Supplementary Fig. S6 . ( d ) Production of TGF-β by pDCs untreated or treated with 1 (pDC/L-CpG) or 10 (pDC/H-CpG) μg ml −1 of ODN. Supernatants were harvested at 72 h after stimulation and assayed for active TGF-β. * P <0.01; Student’s t -test. Full size image The roles of IFN-α, IL-23 and TGF-β in the respective adjuvant and suppressive activities conferred on pDCs by CpG were examined in a skin test assay. In mice lacking a functional type I IFN receptor, the Ifnar −/− pDCs were not amenable to changes in their antigen presentation profile by either lower or higher CpG dosage, nor was GpC capable of any effect in the absence of type I IFN receptor ( Fig. 3a ). In contrast, anti-p19 antibody—but not an anti-TGF-β reagent—added to the pDC cultures during CpG exposure blocked pDC ability to overcome suppression by tolerogenic CD8 + DCs ( Fig. 3c ). The symmetric experiment—using anti-TGF-β on combining pDCs and CD8 − DCs—demonstrated that the induction of suppressive activity by higher-dose CpG was dependent on autocrine TGF-β but independent of p19 ( Fig. 3d ). (As expected [10] , anti-TGF-β also ablated the tolerogenic effect of either GpC dosage in this setting; Supplementary Fig. S7 .) Immunoblot analysis of IDO1 expression proved that adding anti-TGF-β to high-dosage CpG or GpC (and low-dosage GpC as well) would ablate IDO1 protein expression ( Fig. 3 e ). Neutralization of TGF-β did also negate IDO1 functional activity, as measured by tryptophan conversion to kynurenine, regardless of the nature of the tolerogenic ODN ( Fig. 3f ). Not only was the tolerogenic effect of higher-dosage CpG detectable as an induction of functional IDO1, but the conditioned pDCs were also able to bias naive T-cell differentiation towards a Treg phenotype, a likely consequence of the combined effects of tryptophan starvation and tryptophan catabolites [22] . Fluorescence-activated cell sorting analysis of Treg-associated Foxp3 expression in permeabilized CD4 + cells after coculture with CpG- or GpC-conditioned pDCs revealed a higher percentage of Foxp3-expressing CD4 + cells ( Supplementary Fig. S8 ). The specificity of the roles of autocrine IL-23 and TGF-β in the setting of CpG-dependent modulation of pDC function was demonstrated under conditions of in vitro manipulation of pDC function by manoeuvres other than CpG-ODN exposure ( Supplementary Fig. S9a,b ). 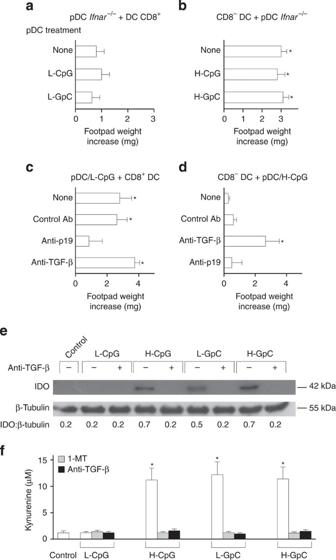Figure 3: Type I IFNs are determinant for the immunomodulatory activities of pDCs treated with CpG or GpC. (a) Splenic CD11c+mPDCA-1+DCs fromIfnar−/−mice were combined with CD8+DCs, pulsed with the P815AB peptide and transferred intravenously into recipient hosts that were assayed at 2 weeks for footpad reactivity to the peptide in saline. Transferred pDCs were either untreated or treated overnight with 1 (pDC/L-CpG) μg ml−1of CpG 1826 or with 1 μg ml−1of the modified, non-CpG ODN 1826 (pDC/L-GpC). Data are mean values±s.d. of four experiments. (b) After overnight exposure to 10 (pDC/H-CpG) μg ml−1CpG or 10 μg ml−1of GpC (pDC/H-GpC), pDCs fromIfnar−/−mice were assayed for suppressive activity of immunogenic peptide presentation by the CD8−DC fraction. The asterisk (*P<0.001; experimental versus control footpads; two-tailed pairedt-test) indicates the occurrence of a positive skin test reaction as a result of immunogenic peptide presentation. Data are mean values±s.d. of four experiments. (c,d) IL-23 and TGF-β dependency of the immunostimulant and immunosuppressive activity of pDCs treated with CpG. Splenic CD11c+DCs were fractionated according to mPDCA-1 or CD8 expression, pulsed with the P815AB peptide and transferred into recipient DBA/2 hosts to be assayed at 2 weeks for skin test reactivity to the eliciting peptide. (c) The pDCs were treated overnight with 1 μg ml−1CpG and cotransferred with a minority fraction of suppressive CD8+DCs. A portion of the pDCs was coexposed to anti-IL-23 p19 (20 μg ml−1) or anti-TGF-β (10 μg ml−1). (d) Alternatively, the pDCs were treated with 10 μg ml−1CpG, with or without anti-TGF-β or anti-IL-23 p19, and cotransferred with a majority fraction of immunogenic CD8−DCs. The asterisks indicate the occurrence of a positive skin test reaction. Data are mean values±s.d. of three experiments. (*P<0.01; experimental versus control footpads; two-tailed pairedt-test). (e) IDO1 protein expression in pDCs treated with low- or high-dose CpG, low- or high-dose GpC, and control or anti-TGF-β (+) antibody was assayed by immunoblot analysis of whole-cell lysates. Blots were stripped and reprobed with anti-β-tubulin. One of three experiments. (f) Functional IDO1 activity was measured in terms of kynurenine levels in supernatants from pDCs treated as above, with either GpC or high-dose CpG. The reference IDO1 inhibitor, 1-methyl-tryptophan (1-MT), was also used in place of anti-TGF-β. Data are means±s.d. of three experiments.P<0.01 (treatment versus control; Student'st-test). Figure 3: Type I IFNs are determinant for the immunomodulatory activities of pDCs treated with CpG or GpC. ( a ) Splenic CD11c + mPDCA-1 + DCs from Ifnar −/− mice were combined with CD8 + DCs, pulsed with the P815AB peptide and transferred intravenously into recipient hosts that were assayed at 2 weeks for footpad reactivity to the peptide in saline. Transferred pDCs were either untreated or treated overnight with 1 (pDC/L-CpG) μg ml −1 of CpG 1826 or with 1 μg ml −1 of the modified, non-CpG ODN 1826 (pDC/L-GpC). Data are mean values±s.d. of four experiments. ( b ) After overnight exposure to 10 (pDC/H-CpG) μg ml −1 CpG or 10 μg ml −1 of GpC (pDC/H-GpC), pDCs from Ifnar −/− mice were assayed for suppressive activity of immunogenic peptide presentation by the CD8 − DC fraction. The asterisk (* P <0.001; experimental versus control footpads; two-tailed paired t -test) indicates the occurrence of a positive skin test reaction as a result of immunogenic peptide presentation. Data are mean values±s.d. of four experiments. ( c , d ) IL-23 and TGF-β dependency of the immunostimulant and immunosuppressive activity of pDCs treated with CpG. Splenic CD11c + DCs were fractionated according to mPDCA-1 or CD8 expression, pulsed with the P815AB peptide and transferred into recipient DBA/2 hosts to be assayed at 2 weeks for skin test reactivity to the eliciting peptide. ( c ) The pDCs were treated overnight with 1 μg ml −1 CpG and cotransferred with a minority fraction of suppressive CD8 + DCs. A portion of the pDCs was coexposed to anti-IL-23 p19 (20 μg ml −1 ) or anti-TGF-β (10 μg ml −1 ). ( d ) Alternatively, the pDCs were treated with 10 μg ml −1 CpG, with or without anti-TGF-β or anti-IL-23 p19, and cotransferred with a majority fraction of immunogenic CD8 − DCs. The asterisks indicate the occurrence of a positive skin test reaction. Data are mean values±s.d. of three experiments. (* P <0.01; experimental versus control footpads; two-tailed paired t -test). ( e ) IDO1 protein expression in pDCs treated with low- or high-dose CpG, low- or high-dose GpC, and control or anti-TGF-β (+) antibody was assayed by immunoblot analysis of whole-cell lysates. Blots were stripped and reprobed with anti-β-tubulin. One of three experiments. ( f ) Functional IDO1 activity was measured in terms of kynurenine levels in supernatants from pDCs treated as above, with either GpC or high-dose CpG. The reference IDO1 inhibitor, 1-methyl-tryptophan (1-MT), was also used in place of anti-TGF-β. Data are means±s.d. of three experiments. P <0.01 (treatment versus control; Student's t -test). Full size image MyD88 is required for CpG adjuvant but not suppressive effects Following preliminary experiments showing that neither lower-dosage nor higher-dosage CpG affects Tlr9 transcription (nor does either GpC dosage; Supplementary Fig. S10 ), we examined the role of the essential TLR adaptors MyD88 (myeloid differentiating factor 88) and TRIF (Toll/IL-1 receptor domain-containing adaptor inducing IFN-β) in pDC conditioning by low- or high-dose CpG. In a first set of experiments, by assaying skin test reactivity to the HY peptide and using genetically deficient ( Tlr9 −/− or Myd88 −/− ) donors of pDCs, we confirmed that the immunostimulant effect of a lower CpG dosage required TLR9 and MyD88 signalling. We examined the effects of CpG-conditioned pDCs admixed with a minority fraction of tolerogenic CD8 + DCs ( Fig. 4a ). In the reciprocal combination (that is, on admixing immunogenic CD8 − DCs with 5% CpG-conditioned pDCs), the suppressive effect of the higher CpG dosage required TLR9 signalling but was independent of MyD88 ( Fig. 4b ). (As expected [10] , under the same experimental conditions, the tolerogenic effects of GpC required neither TLR9 nor MyD88, Fig. 4b .) IDO1 functional activity was initiated by high-dose CpG, in wild-type and Myd88 −/− mice but not in Tlr9 −/− pDCs ( Fig. 4 c ). In contrast, the GpC-ODN was effective in inducing functional IDO1 under conditions of either MyD88 or TLR9 deficiency ( Fig.4c ). Again, in all of these experiments the nc-ODN lacked biological activity ( Fig. 4a–c ). p19-encoding Il23a was induced transcriptionally by low-dose CpG in wild-type but not Tlr9 −/− or Myd88 −/− mice, whereas Tgfb1 was induced by the higher CpG dosage in wild-type and Myd88 −/− mice but not in Tlr9 −/− mice. This was in marked contrast with the pattern of TGF-β production by GpC ( Supplementary Fig. S11a,c ). Direct comparison of IL-23 and TGF-β productions in wild-type and Myd88 −/− mice treated with 1 or 10 μg ml −1 CpG-ODN 1826 for 24 h confirmed that IL-23 production was selectively affected by MyD88 deficiency ( Supplementary Fig. S11b ). In addition, using a different method of TGF-β induction, namely tolerogenic CTLA-4–Ig, cytokine production was unaffected by genetic deficiency of TLR9 or MyD88 ( Supplementary Fig. S12 ). 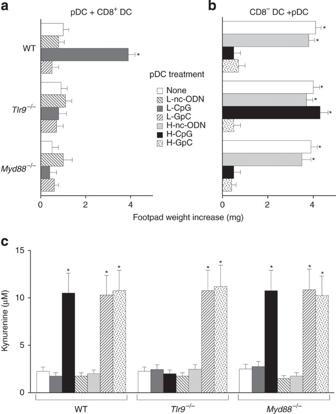Figure 4: TLR9–MyD88 dependency of CpG adjuvant effect. (a) Induction of skin test reactivity by CpG requires TLR9 as well as MyD88 signalling in pDCs. Wild-type (WT) C57BL/6 pDCs were treated overnight with 1 μg ml−1CpG (L-CpG), nc-ODN (L-nc-ODN) or GpC (L-GpC), pulsed with the HY peptide, and cotransferred with a minority fraction of suppressive CD8+DCs. Parallel groups included pDCs fromTlr9−/−orMyd88−/−mice. Skin test reactivity to the eliciting peptide was measured at 2 weeks. (b) Suppression of skin test reactivity by CpG requires TLR9 but not MyD88 signalling, whereas the suppressive effect of GpC occurs independently of TLR9 and MyD88. pDCs from WT or genetically deficient mice were treated with 10 μg ml−1CpG (H-CpG), nc-ODN (H-nc-ODN) or GpC (H-GpC), and cotransferred with a majority fraction of immunogenic CD8−DCs. In bothaandb, the asterisks indicate the occurrence of a positive skin test reaction (*P<0.01; experimental versus control footpads; two-tailed pairedt-test), and data are mean values±s.d. of three experiments. (c) IDO1 functional activity is induced by high-dose CpG inMyd88−/−but notTlr9−/−mice, and by either GpC dosage in bothMyd88−/−andTlr9−/−mice. Functional IDO1 activity was measured in terms of kynurenine production by pDCs treated with either dosage of CpG, nc-ODN or GpC. Data are means±s.d. of three experiments.P<0.01 (treatment versus none; Student'st-test). Figure 4: TLR9–MyD88 dependency of CpG adjuvant effect. ( a ) Induction of skin test reactivity by CpG requires TLR9 as well as MyD88 signalling in pDCs. Wild-type (WT) C57BL/6 pDCs were treated overnight with 1 μg ml −1 CpG (L-CpG), nc-ODN (L-nc-ODN) or GpC (L-GpC), pulsed with the HY peptide, and cotransferred with a minority fraction of suppressive CD8 + DCs. Parallel groups included pDCs from Tlr9 −/− or Myd88 −/− mice. Skin test reactivity to the eliciting peptide was measured at 2 weeks. ( b ) Suppression of skin test reactivity by CpG requires TLR9 but not MyD88 signalling, whereas the suppressive effect of GpC occurs independently of TLR9 and MyD88. pDCs from WT or genetically deficient mice were treated with 10 μg ml −1 CpG (H-CpG), nc-ODN (H-nc-ODN) or GpC (H-GpC), and cotransferred with a majority fraction of immunogenic CD8 − DCs. In both a and b , the asterisks indicate the occurrence of a positive skin test reaction (* P <0.01; experimental versus control footpads; two-tailed paired t -test), and data are mean values±s.d. of three experiments. ( c ) IDO1 functional activity is induced by high-dose CpG in Myd88 −/− but not Tlr9 −/− mice, and by either GpC dosage in both Myd88 −/− and Tlr9 −/− mice. Functional IDO1 activity was measured in terms of kynurenine production by pDCs treated with either dosage of CpG, nc-ODN or GpC. Data are means±s.d. of three experiments. P <0.01 (treatment versus none; Student's t -test). Full size image CpG-suppressive effects depend on TRIF but not TLR3 or TLR4 In a second set of experiments, by examining skin test reactivity to the HY peptide as modulated by pDCs lacking TRIF-encoding Ticam1 , Tlr3 or Tlr4 , we obtained evidence that the tolerogenic effect of a higher CpG dosage, and of GpC as well, required TRIF but neither TLR3 nor TLR4, with which TRIF typically associates ( Fig. 5a ). Tgfb1 expression was induced by higher-dose CpG (or GpC at either dosage) in Tlr3 −/− or Tlr4 −/− mice but not in Ticam1 −/− pDCs, lacking TRIF ( Supplementary Fig. S13 ). IDO1 functional activity, when triggered by high-dose CpG, or GpC, was demonstrable in pDCs from TLR3- or TLR4- but not TRIF-deficient mice ( Fig. 5b ). 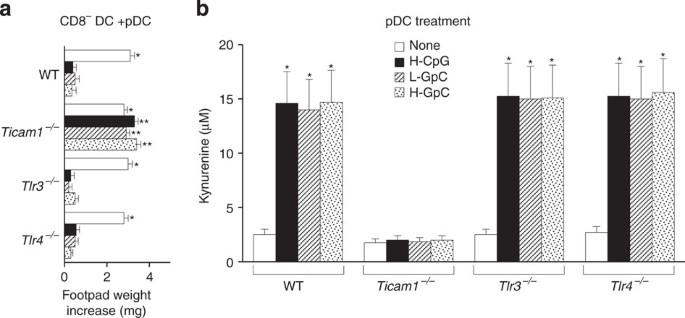Figure 5: Tolerogenesis by CpG and GpC requires TRIF but not TLR3 or TLR4 signalling. (a) pDCs from WT or genetically deficient mice were treated with 10 μg ml−1CpG (H-CpG), or with 1 or 10 μg ml−1GpC (L-GpC and H-GpC, respectively) and cotransferred with a majority fraction of spontaneously immunogenic CD8−DCs. The asterisks indicate the occurrence of a positive skin test reaction (*P<0.01 and **P<0.001; experimental versus control footpads; two-tailed pairedt-test), and data are mean values±s.d. of three experiments. (b) IDO1 functional activity is induced by high-dose CpG and by both low- and high-dose GpC administrations toTlr3−/−orTlr4−/−but notTicam1−/−mice. Enzyme activity was measured in terms of kynurenine production by the pDCs treated with CpG or GpC. Data are means±s.d. of three experiments.P<0.01 (treatment versus none; Student'st-test). Figure 5: Tolerogenesis by CpG and GpC requires TRIF but not TLR3 or TLR4 signalling. ( a ) pDCs from WT or genetically deficient mice were treated with 10 μg ml −1 CpG (H-CpG), or with 1 or 10 μg ml −1 GpC (L-GpC and H-GpC, respectively) and cotransferred with a majority fraction of spontaneously immunogenic CD8 − DCs. The asterisks indicate the occurrence of a positive skin test reaction (* P <0.01 and ** P <0.001; experimental versus control footpads; two-tailed paired t -test), and data are mean values±s.d. of three experiments. ( b ) IDO1 functional activity is induced by high-dose CpG and by both low- and high-dose GpC administrations to Tlr3 −/− or Tlr4 −/− but not Ticam1 −/− mice. Enzyme activity was measured in terms of kynurenine production by the pDCs treated with CpG or GpC. Data are means±s.d. of three experiments. P <0.01 (treatment versus none; Student's t -test). Full size image Next, we examined cytokine (IL-6, IL-10, IL-23, IFN-α, IFN-γ, TGF-β, IL-12 p40, IL-12 p70 and tumour-necrosis factor (TNF)-α) production in wild-type, Tlr9 −/− , Myd88 −/− or Ticam −/− pDCs exposed to high-dose or low-dose CpG ( Supplementary Fig. S14a ). In response to high-dose CpG, the production of IFN-α required TLR9- and TRIF-dependent signalling, whereas low-dose CpG induced IL-23 and IFN-α via TLR9 and MyD88. Wild-type, Tlr9 −/− , Myd88 −/− or Ticam −/− pDCs exposed to high-dose or low-dose CpG were also assayed by immunoblotting for IDO1 protein expression ( Supplementary Fig. S14b ), demonstrating the need for functional TLR9 and TRIF. Induction of IFN-α, TGF-β and functional IDO was dependent on the TRIF competence of GpC-treated pDCs but required neither TLR9 nor MyD88 ( Supplementary Fig. S14a,b ). Direct association of TRIF with TLR9 could be demonstrated in an HEK293 cell line that stably expressed mouse TLR9 fused, at the carboxyl terminus, with the influenza hemagglutinin tag ( Supplementary Fig. S15 ). TRAF proteins are required for both activities of CpG TNF-receptor-associated factors (TRAFs) are intracellular proteins that bind the cytoplasmic portion of TNF receptors and mediate downstream signalling. The six known TRAF proteins (TRAF1–6) have overlapping yet distinct roles in controlling immune responses as well as cellular processes [23] . TRAF3 is one of the most enigmatic members in the TRAF family and has been identified to perform apparently distinct roles. Recent studies suggest that nuclear factor κB-inducing kinase (crucial in noncanonical NF-κB signalling) is suppressed through constitutive proteasome-mediated degradation regulated by TRAF2 and TRAF3 (ref. 24 ). In contrast, TRAF6 contributes to CD40-mediated activation of NF-κB, stress-activated protein kinases and other signalling molecules [25] . We investigated the possible involvement of the two TRAF proteins in the P815AB skin test model system by siRNA technology. TRAF3-specific siRNA—but not TRAF6-specific siRNA—added to the pDC cultures during CpG exposure blocked pDC ability to overcome suppression by tolerogenic CD8 + DCs ( Supplementary Fig. S16a ). In the other setting—using siRNA on combining pDCs and CD8 − DCs—we found that the induction of suppressive activity by higher-dose CpG was dependent on TRAF6 but independent of TRAF3 ( Supplementary Fig. S16b,c ). Dominance of canonical and noncanonical NF-κB signalling IDO1 expression is contingent on the noncanonical pathway of NF-κB activation [19] , [26] , [27] . Molecular dissection of NF-κB activation has shown that NF-κB can be induced by the so-called canonical (classical; IκB kinase (IKK)β-dependent) and noncanonical (alternative; IKKα-dependent) signalling pathways, leading to distinct patterns in the individual NF-κB subunits that are activated and the downstream genetic responses that are induced. Both the Tgfb1 and Ido1 promoters contain putative noncanonical NF-κB-binding sites recognized by noncanonical p52/RelB dimers [17] , [21] , [26] , [27] . Much like CD40 ligation [27] , in IDO1 + pDCs, triggering of TLR9 can activate both the IKKα- and IKKβ-mediated pathways [28] . Using immunoblot analysis, we examined CpG at 1 or 10 μg ml −1 for possible activation of canonical and noncanonical NF-κB pathways ( Fig. 6a ). Lower-dose CpG activated phosphorylation of both IKKα and IKKβ, and 10 μg ml −1 CpG activated higher-level phosphorylation of only IKKα. We used ELISA to determine the relative amounts of canonical p65 and noncanonical p52 in wild-type or genetically deficient pDCs treated with CpG. We found a progressive increase of p65 in wild-type and Ticam1 −/− , but neither Tlr9 −/− nor Myd88 −/− , pDCs ( Fig. 6b ). In parallel, p52—as induced by the higher CpG dosage—increased over time and to comparable extents in control and MyD88-competent mice, but not in TLR9- or TRIF-deficient pDCs ( Fig. 6c ). In parallel gene-silencing experiments, we found that p65 activation by lower-dose CpG required TRAF3 but not TRAF6 ( Fig. 6b ), whereas p52 activation by higher CpG treatment required TRAF6 but not TRAF3 ( Fig. 6c ). In gene-silencing experiments in vivo , IKKα but not IKKβ was required for high-dose CpG to confer tolerogenic properties on pDCs in a skin test assay ( Supplementary Fig. S17a,b ). 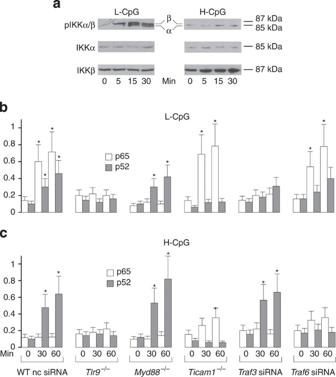Figure 6: Respective dominance of MyD88/canonical and TRIF/noncanonical NF-κB signalling pathways as induced by immunostimulant and immunosuppressive CpG. (a) Low-dose CpG activates phosphorylation of IKKα and IKKβ whereas higher-dose CpG activates phosphorylation of IKKα. pDCs were treated with 1 or 10 μg ml−1CpG for different times and immunoblots of cell lysates were probed with anti-pIKKα/β followed by anti-IKKα or anti-IKKβ. One experiment representative of three. ELISA measurements were used to determine the relative amounts (A450) of p65 and p52 in pDCs treated with low-dose CpG (b) or high-dose CpG (c) as above for different times. Nuclear extracts were obtained from cells of WT or genetically deficient mice. Data are means±s.d. of three experiments. *P<0.05–0.01 (treatment versus respective time 0 control; Student’st-test). Figure 6: Respective dominance of MyD88/canonical and TRIF/noncanonical NF-κB signalling pathways as induced by immunostimulant and immunosuppressive CpG. ( a ) Low-dose CpG activates phosphorylation of IKKα and IKKβ whereas higher-dose CpG activates phosphorylation of IKKα. pDCs were treated with 1 or 10 μg ml −1 CpG for different times and immunoblots of cell lysates were probed with anti-pIKKα/β followed by anti-IKKα or anti-IKKβ. One experiment representative of three. ELISA measurements were used to determine the relative amounts ( A 450 ) of p65 and p52 in pDCs treated with low-dose CpG ( b ) or high-dose CpG ( c ) as above for different times. Nuclear extracts were obtained from cells of WT or genetically deficient mice. Data are means±s.d. of three experiments. * P <0.05–0.01 (treatment versus respective time 0 control; Student’s t -test). Full size image Overall, it would appear that lower dosages of CpG-ODN will result in limited yet coexistent activation of IKKβ and IKKα, but higher dosages will selectively result in high-level noncanonical activation (in the relative absence of canonical signalling, which is, in fact, actively suppressed by the former). This might explain the coexistence of IL-23 and IFN-α under lower CpG-ODN treatment conditions and the great preponderance of TGF-β found on treating pDCs with higher CpG-ODN concentrations. Stimulation and suppression depend on IRF7 and IRF3, respectively Expression and function of type I IFNs can be regulated by IFN regulatory factor (IRF)3 and 7, typically activated by the triggering of signalling cascades from TLRs that recognize pathogenic nucleic acids. TLR9 signalling in pDCs activates the MyD88-dependent canonical NF-κB pathway and the IRF7-dependent IFN pathway [29] . We investigated whether the effects of lower and higher CpG dosages are contingent on IRFs. pDCs, either untreated or treated with lower-dose CpG, were used in combination with a minority fraction of tolerogenic CD8 + DCs in a skin test assay. A portion of the pDCs had been transfected with negative control, IRF3-specific, or IRF7-specific siRNA ( Supplementary Fig. S18a ). In parallel, pDCs, treated with high-dose CpG, were cotransferred with a majority fraction of immunogenic CD8 − DCs. A portion of the pDCs had likewise been transfected with negative control, or Irf3 - or Irf7 -targeting siRNA ( Supplementary Fig. S18b ). The results provided evidence for the dependence of the stimulant effect on IRF7, as well as for IRF3, as a required component of the tolerogenic circuit. In addition, high-dose CpG induced nuclear translocation of IRF3 in pDCs from wild-type and Myd88 −/− , but not Ticam1 −/− , mice ( Supplementary Fig. S18c ). Finally, high-dose CpG induced Tgfb1 and IDO1 protein expression in the absence of functional IRF7, yet both effects required IRF3 ( Supplementary Fig. S18d–f ). Although the mechanisms whereby IRF3 contributes to Tgfb1 transcription are unclear, this might be compatible with the notion that TRIF-dependent signalling activates multiple transcription factors, including IRF3, NF-κB and AP-1, leading to induction of type I IFNs and other cytokines [30] , [31] , likely via an IRF3–IFN-β–STAT1 pathway, in response to TLR activation [32] . This interpretation is consistent with the need for a functional type I IFN receptor in the higher-dose-suppressive effect of CpG ( Fig. 3b ). In addition, it should be noted that the Tgfb1 promoter contains, itself, a putative consensus motif (5′-AAAGGAAA-3′; from −1,412 to −1,405 bp, relative to transcription start site) for binding IRF3. Differential IDO induction and cytokine production in human DCs We investigated the possible effects of CpG conditioning on human Flt3L-derived DCs (FL-DCs) by analysing IDO expression and cytokine production. Following preliminary experiments suggesting dichotomic effects of 0.3 μg ml −1 (low-dose) and 3 μg ml −1 (high-dose) CpG 2006, human purified FL-DCs were exposed to either CpG-ODN concentration and were then used in immunoblotting ( Fig. 7a ) and cytokine production experiments ( Fig. 7b ). The human TLR9-recognizing ODN sequence containing the CpG motif strongly induced IDO1 expression and TGF-β production only when used at 3 μg ml −1 . In contrast, IL-23 production was only observed with the lower CpG concentration. Co-immunoprecipitation experiments showed that the high-dose CpG effect was associated with TLR9’s recruitment of TRIF and TRAF6, whereas the lower-dose effect relied on the association of TLR9 with MYD88 and TRAF3 ( Fig. 7c ). These data are in line with a previous report showing that both CpG-A and CpG-C ODN-activated human pDCs will similarly induce the generation of CD4 + CD25 + Treg cells with strong immune-suppressive function, demonstrating that TLR9 stimulation can promote pDC-mediated generation of CD4 + CD25 + Treg cells [33] . 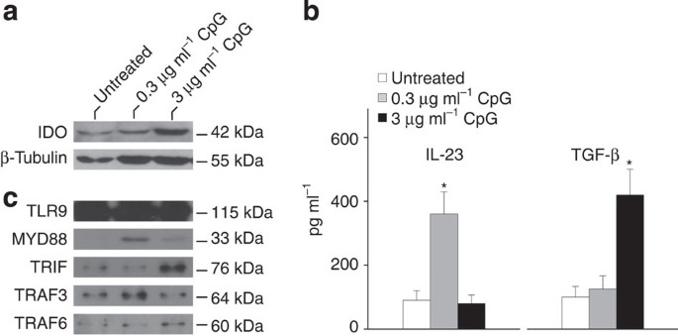Figure 7: Effect of CpG treatment on human DCs. (a) IDO protein expression was analysed in FL-DCs, either untreated or treated with 0.3 or 3 μg ml−1CpG. (b) FL-DCs were assayed for IL-23 and TGF-β release after 0.3 or 3 μg ml−1CpG exposure. Data are means±s.d. from four experiments. *P<0.05; Student’st-test. (c) TLR9 associates with MYD88 and TRAF3 upon stimulation with 0.3 μg ml−1CpG, but with TRIF and TRAF6 after stimulation with 3 μg ml−1CpG. One experiment representative of several. Figure 7: Effect of CpG treatment on human DCs. ( a ) IDO protein expression was analysed in FL-DCs, either untreated or treated with 0.3 or 3 μg ml −1 CpG. ( b ) FL-DCs were assayed for IL-23 and TGF-β release after 0.3 or 3 μg ml −1 CpG exposure. Data are means±s.d. from four experiments. * P <0.05; Student’s t -test. ( c ) TLR9 associates with MYD88 and TRAF3 upon stimulation with 0.3 μg ml −1 CpG, but with TRIF and TRAF6 after stimulation with 3 μg ml −1 CpG. One experiment representative of several. Full size image pDCs treated with high-dose CpG prevent airway inflammation We investigated the effect of in vitro conditioning of pDCs with high-dose CpG on the induction of airway inflammation upon cell transfer onto recipient hosts. Mice were sensitized and challenged by ovalbumin (OVA) to induce airway inflammation. OVA-pulsed splenic pDCs, either untreated or treated overnight with 10 μg ml −1 CpG-ODN, were injected intravenously into mice before subjecting recipients to a fully immunogenic asthma protocol, consisting of two intraperitoneal injection of OVA in alum, followed by an intranasal OVA challenge. Mice on untreated wild-type, Myd88 −/− or Ticam1 −/− pDC treatment developed eosinophilic airway inflammation, as demonstrated by histology of lung sections ( Supplementary Fig. S19a ), and circulating IgE and Th2 cytokines ( Supplementary Fig. S19b ). In contrast, administration of OVA-pulsed wild-type and Myd88 −/− , but not Ticam1 −/− , pDCs treated with high-dose CpG-ODN strongly opposed allergy development ( Supplementary Fig. S19a,b ). Thus TRIF, but not MyD88, is necessary to mediate the tolerogenic effect of pDCs exposed in vitro to CpG in an allergic airway model system. CpG protection against ABPA in vivo requires TLR9 and TRIF Allergic bronchopulmonary aspergillosis (ABPA) is a Th2-sustained allergic condition of the lung in humans. Experimental models of the disease have been used to demonstrate a pivotal role for Treg cells [19] , [26] , pDCs [34] and tryptophan catabolism [35] , [36] in protecting mice from allergic airway inflammation. We evaluated any TLR9, MyD88 and TRIF dependency of the effects of CpG on the hypersensitivity response to Aspergillus antigens in the mouse lung. Bronchial colonization of Aspergillus fumigatus was established after the elicitation of a strong Th2 reactivity, and the animals (either wild-type or lacking TLR9, MyD88 or TRIF) were treated with CpG-ODN 1826 (30 μg per mouse twice, in concomitance with allergen) to be assessed for parameters of allergic airway inflammation. At 1 week of colonization, the number of eosinophils in the bronchoalveolar lavage (BAL) fluid and circulating IgE antibody—both indicative of A. fumigatus respiratory allergy [35] —were decreased by CpG treatment relative to mice either untreated or lacking TLR9 or TRIF. In the latter mice—and most prominently in TRIF-deficient mice—histopathology confirmed the presence of extensive peribronchial infiltrates of mononuclear cells and eosinophils, globet cell hyperplasia and mucus deposition in the airways ( Fig. 8a ). 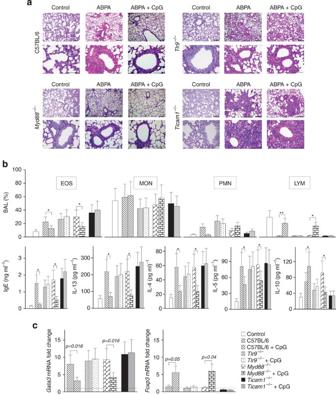Figure 8: Effect of CpG treatment on allergic airway inflammation and requirement for TRIF but not MyD88 signalling. Bronchial colonization withA. fumigatuswas established in wild-type,Tlr9−/−,Myd88−/−andTicam1−/−Th2-primed mice with or without CpG treatment, to be assayed forA. fumigatusallergy at 1 week. Unsensitized, uncolonized wild-type mice (control) and genetically deficient mice (indicated) were present in all assays, and so were sensitized and colonized mice of all genotypes on CpG treatment. Control littermates were included in individual experiments to check for nonspecific effects of each genetic manipulation, and none were found. (a) Paraffin-embedded lung sections were stained with periodic acid-Schiff to visualize mucine, goblet cells and inflammatory cells. Data are representative of three independent experiments. Upper panels, scale bar, 200 μm; and lower panels, scale bar, 100 μm. CpG treatment alone was indistinguishable from control. (b) The abundance of eosinophils (eos), monocytes (mon), polymorphonucleates (pmn) and lymphocytes (lym) was assessed in BAL fluid. IgE antibodies were determined in sera, and secreted cytokines were measured in BAL fluid. Control, naïve C57BL/6 mice. Data are mean±s.d. of three experiments. *P<0.05 and **P<0.005; Student’st-test. (c)Gata3andFoxp3transcripts were evaluated in CD4+T cells from thoracic lymph nodes. Sorted CD4+lymphocytes (5 × 105ml−1) were activated with soluble antibodies to CD3 for 24 h.Gata3andFoxp3mRNAs were quantified by real-time PCR usingGapdhnormalization. Data (mean±s.d. of three (Foxp3) or four (Gata3) experiments) are presented as normalized transcript expression in the samples relative to normalized transcript expression in the control culture (cells from naïve mice of the respective genotype; that is, fold change =1, dotted line). Figure 8: Effect of CpG treatment on allergic airway inflammation and requirement for TRIF but not MyD88 signalling. Bronchial colonization with A. fumigatus was established in wild-type, Tlr9 −/− , Myd88 −/− and Ticam1 −/− Th2-primed mice with or without CpG treatment, to be assayed for A. fumigatus allergy at 1 week. Unsensitized, uncolonized wild-type mice (control) and genetically deficient mice (indicated) were present in all assays, and so were sensitized and colonized mice of all genotypes on CpG treatment. Control littermates were included in individual experiments to check for nonspecific effects of each genetic manipulation, and none were found. ( a ) Paraffin-embedded lung sections were stained with periodic acid-Schiff to visualize mucine, goblet cells and inflammatory cells. Data are representative of three independent experiments. Upper panels, scale bar, 200 μm; and lower panels, scale bar, 100 μm. CpG treatment alone was indistinguishable from control. ( b ) The abundance of eosinophils (eos), monocytes (mon), polymorphonucleates (pmn) and lymphocytes (lym) was assessed in BAL fluid. IgE antibodies were determined in sera, and secreted cytokines were measured in BAL fluid. Control, naïve C57BL/6 mice. Data are mean±s.d. of three experiments. * P <0.05 and ** P <0.005; Student’s t -test. ( c ) Gata3 and Foxp3 transcripts were evaluated in CD4 + T cells from thoracic lymph nodes. Sorted CD4 + lymphocytes (5 × 10 5 ml −1 ) were activated with soluble antibodies to CD3 for 24 h. Gata3 and Foxp3 mRNAs were quantified by real-time PCR using Gapdh normalization. Data (mean±s.d. of three ( Foxp3 ) or four ( Gata3 ) experiments) are presented as normalized transcript expression in the samples relative to normalized transcript expression in the control culture (cells from naïve mice of the respective genotype; that is, fold change =1, dotted line). Full size image The analysis of the patterns of Th1, Th2 and Treg-associated cytokine production in BAL fluid showed a profile typical of Aspergillus allergy in mice either untreated or treated with CpG but lacking TLR9 or TRIF, characterized by a dominant production of IL-5, IL-4 and IL-13, a key mediator in inflammatory processes in the asthmatic lung ( Fig. 8b ). Again, the Th2-dependent allergic phenotype was greatly attenuated by CpG, which enhanced the production of IL-10, a marker of protective Treg activity in Aspergillus allergy [36] ( Fig. 8b ). The cytokine pattern was consistent with PCR assessment of Gata3 and Foxp3 transcripts in thoracic lymph node CD4 + T cells ( Fig. 8c ). The Th2 transcription factor GATA3 was downregulated together with an enhanced expression of the Treg lineage specification factor, Foxp3, in mice on CpG treatment expressing TLR9 and TRIF. These data demonstrate that CpG downregulates exacerbating Th2 responses in ABPA by inhibiting the expansion and activation of Th2 cells, and upregulates Foxp3 expression via mechanisms that require TLR9 and TRIF but not MyD88. It is interesting to note that in the model of ABPA, resident pDCs will confer protective tolerance to Aspergillus [37] and that protection can be adoptively transferred by pulsed DCs that exploit anti-inflammatory, IDO-dependent pathways [38] , involving Treg cell generation [39] . CpG-ODNs have potent immunostimulatory effects on pDCs through TLR9 recognition and signalling [40] . However, immunosuppression occurs after repeated or systemic CpG-ODN administration, which, triggered by TLR9 signalling [41] , may [6] or may not [8] require autocrine IFNs. In this paper, we provide evidence that tolerogenic signalling via TLR9 (a) occurs as a function of not only route but also dose of CpG administration; (b) requires physical association with the adaptor TRIF and is independent of TLR3, TLR4 and MyD88; (c) results in the IRF3-dependent induction of type I IFNs, TGF-β and functional IDO1, all of which contribute to tolerogenesis, likely via a pDCs–Treg axis [12] . Moreover our data indicate that (d) immunostimulant activity by lower-dose CpG requires, instead, the TLR9–MyD88 pathway as well as production of the proinflammatory cytokine IL-23; (e) genetic deficiency of MyD88 negates functional effects by lower-dose CpG, implying that direction of response depends upon ligand concentration, which likely affects the affinity with which TLR9 recruits downstream adaptor and signalling molecules, including TRAF3 and TRAF6; (f) the protective effects of CpG in experimental allergy in vivo require a TLR9–TRIF circuit but not MyD88-dependent events. Not secondarily, we also confirmed that (g) a non-CpG ODN with two GpC motifs is exclusively immunosuppressive in the same setting, an effect we have recently demonstrated not to require TLR9 and be, in fact, contingent on TLR7- and TRIF-dependent signalling events [10] . As a corollary, a role, per se , of the phosphorothioate backbone in the TLR7 (GpC-dependent) and TLR9 (higher-dose CpG-dependent) pathways of tolerogenesis is ruled out by the stimulatory effect of lower-dose CpG on the same backbone, which is in line with the dual effects both of CpG on a phosphodiester backbone and of bacterial DNA. Finally, (h) differential IDO induction and cytokine production by low- versus high-dose CpG could also be documented in human DCs. The TLR4 pathway employs signalling through two distinct adaptors, MyD88 and TRIF, and there is evidence that some CpG-ODNs may also require a second receptor or cofactor to signal in addition to TLR9 (ref. 42 ). Although the molecular basis of TLR4 signalling transition in response to endotoxin is unclear [43] , evidence suggests that the MyD88 and TRIF pathways are temporally segregated, nonetheless influencing each other [44] . Early signalling through MyD88 leads to phosphorylation-mediated degradation of IκBα, nuclear translocation of NF-κB p65/p50 heterodimers and transcription of proinflammatory genes such as TNFA , IL1B , IL12B and IL6 . Later in time, as endotoxin concentrations increase, and owing to a prevailing TRIF-dependent signalling and plasticity of NF-κB function, accumulating p50/p50 NF-κB homodimers trigger the transcription of genes like IL10 , TGFB1 and COX2 (refs 43 , 45 ). This could be seen as a form of ‘protective’ [35] or ‘infectious’ [21] tolerance, whereby exaggerated inflammatory responses are avoided via the rapid onset of cell refractoriness to sustained stimulation and the spread of a tolerant state from one cell type to another. Seen in this light, both the selective induction of immunosuppression in the spleen by systemic CpG-ODN [7] , [8] and the duality of its effects as a function of local concentrations in the microenvironment might reflect a negative feedback mechanism in order to avoid hyperinflammatory responses [27] , [45] , [46] . TLR9 modulation of IDO1 is effective not only in the prevention and treatment of animal models of autoimmune [13] and allergic disorders [4] , [6] , [8] , but also in maintaining a physiological state of protective tolerance to ubiquitous fungal aeroantigens [36] . ABPA is a Th2-dependent hypersensitivity lung disease due to bronchial colonization of A. fumigatus that affects 1–2% of asthmatic and 7–9% of cystic fibrosis patients. Although the organism can cause allergic disease in otherwise healthy individuals and devastating disease in the immunosuppressed, ABPA is a hypersensitivity response to Aspergillus antigens in the lung and is distinct from other forms of Aspergillus pulmonary disease. In an experimental model of ABPA, in which the combined effects of Treg cells, pDCs and tryptophan catabolism mediate protection, we have previously found that dexamethasone inhibited Th2 responses and allergy, and induced Foxp3 expression in CD4 + T cells via mechanisms dependent on tryptophan catabolism [26] . Here, using the same model system, we found that the beneficial activity of CpG immunotherapy involves the TLR9–TRIF pathway, independently of MyD88. In conclusion, our results demonstrate the occurrence of a functional TLR9–IDO1 axis involving type I IFNs and TGF-β. Although the molecular basis of the switch in TLR9 signalling outcomes from an inflammatory MyD88-dependent to an immunosuppressive TRIF-dependent effect remains elusive, our study shows that CpG ODN-induced immune stimulation is characterized by a bell-shaped dose–response correlation, that is, only intermediate but not high doses of CpG induce effects typically associated with immune activation. In contrast, higher dosages trigger TLR9- and IDO1-dependent tolerogenesis, which abrogates the stimulatory effects and relies on TRIF and the noncanonical NF-κB signalling pathway as well as on TGF-β production, which may further exploit IDO1 as a signalling protein in a feedforward loop involving the stable conditioning of pDCs towards a regulatory phenotype [12] . These data may have an impact on novel CpG-based therapeutic approaches in the context of antitumor and vaccination strategies, including siRNA delivery approaches targeting phagocytic cells through an siRNA conjugated to a TLR9 ligand [1] . These studies may also lead to innovative means of treating autoimmune and allergic inflammation. Mice Eight- to 10-week-old female DBA/2J (H-2 d ), C57BL/6 (H-2 b ) and 129 Sv/Ev (H-2 b ) mice were obtained from Charles River Breeding Laboratories. Female mice deficient for the IFN-α/β receptor ( Ifnar −/− ), on a 129 Sv/Ev background, were generated as described [26] . Mice homozygous for the TLR3 ( Tlr3 −/− ), TLR4 ( Tlr4 −/− ), TLR9 ( Tlr9 −/− ), MyD88 ( Myd88 −/− ) or TRIF ( Ticam1 −/− )-targeted mutation raised on the C57BL/6 background were as described [13] and were bred at the breeding facilities of the University of Perugia. All in vivo studies were in compliance with National (Italian Parliament DL 116/92) and Perugia University Animal Care and Use Committee guidelines. DC purification and treatments These procedures have been described in previous publications [47] , [48] . Briefly, splenic DCs were purified by magnetic-activated sorting using CD11c MicroBeads and MidiMacs (Miltenyi Biotec, Bergisch Gladbach, Germany), in the presence of EDTA to disrupt DC–T-cell complexes. Cells were >99% CD11c + , >99% MHC I-A + , >98% B7-2 + , <0.1% CD3 + , and appeared to consist of 90–95% CD8 − , 5–10% CD8 + and ~5% mPDCA-1 + cells. For positive selection of mPDCA-1 + DCs (6), CD11c + cells were fractioned using mPDCA-1 MicroBeads (Miltenyi Biotec). More than 95% of the mPDCA-1 + cells were stained by 120G8. For negative selection of CD8 − DCs, CD11c + cells were fractioned by means of CD8α MicroBeads (Miltenyi Biotec). The CD8 − fraction was ~45% CD4 + and typically contained <0.5% contaminating CD8 + cells. Less than 5% CD8 − DCs expressed the 120G8 marker. All endotoxin-free CpG-ODNs either on a phosphorothioate (ODN 1826 (5′-tccatga cg ttcctga cg tt-3′), ODN 1826 negative control (nc-ODN; 5′-tccatgatattcctgatatt-3′), ODN 1826 non-CpG control (GpC; 5′-tccataa gc ttcctga gc tt-3′), ODN 2006 (5′-t cg t cg ttttgt cg ttttgt cg tt-3′)) or on a phosphodiester backbone (CpG-A (5-TCCATGA CG TTCCTGA CG TT-3)) were purchased from Invitrogen Life Technologies. (Lowercase letters in ODN sequences refer to nucleotides for which the 3′ internucleotide linkage is phosphorothioate-modified; endotoxin contamination, when measured by the Limulus assay (Sigma), was negligible in all ODN preparations.) pDCs were treated in vitro with 1 or 10 μg of CpG-ODN 1826 or the control ODNs. siRNA synthesis and transfection These procedures, performed according to standard methodologies, are described in full in Supplementary Methods . Immunization and skin test assay The skin test assay we have been using measures class I-restricted responses to synthetic peptides (H-2L d –restricted P815AB.35-43 [LPYLGWLVF] and H-2D b –restricted HY [WMHHNMDLI]). Following intravenous transfer of peptide-pulsed DCs, the response to intrafootpad challenge with the soluble peptide was measured, as described previously in detail [20] , [26] and also elucidated in Supplementary Methods . Kynurenine assay IDO1 functional activity was measured in vitro in terms of the ability of DCs to metabolize tryptophan to kynurenine, whose concentrations were measured by HPLC, as described previously [26] , [48] . Immunoblot and ELISA analyses These procedures, performed according to standard methodologies, are described in full in Supplementary Methods . PCR assay PCR assessment of Gata3 and Foxp3 transcripts in thoracic lymph node CD4 + T cells was described [26] , [35] . Human FL-DC preparation and immunoprecipitation Human mature FL-DCs were obtained from peripheral blood mononuclear cells (PBMCs). Briefly, PBMCs were separated from whole blood of healthy donors by centrifugation through a density gradient of Ficoll–Paque (GE Healthcare). Whole blood was layered onto a sterile aqueous medium containing Ficoll at a predetermined density of 1.077 g ml −1 at 25 °C. Gentle centrifugation at room temperature resulted in the separation of PBMCs at the blood/Ficoll interface, with the other white blood cells and red blood cells passing through the interface and accumulating at the bottom of the tube. FL-DCs were obtained from purified CD14 + monocytes by culturing cells in Iscove-modified medium for 7 days in the presence of 50 ng ml −1 of human FLT3L (Peprotech). The resulting FL-DCs were washed and cultured for 18 h with 0.3 or 3 μg ml −1 of CpG-ODN 2006 (5′-TCGTCGTTTTGTCGTTTTGTCGTT-3′). Supernatants were then analysed for cytokine production (IL-23 and TGF-β; Promega) and cell lysates for IDO expression by western blotting using an anti-human IDO reagent (Millipore). FACS analysis revealed that the FL-DCs were CD123 + CD11c low BDCA2 + and BDCA4 + . For immunoprecipitation, FL-DCs (100 × 10 6 cells per sample) were stimulated for 30 min with low-dose (0.3 μg ml −1 ) or high-dose (3 μg ml −1 ) CpG 2006, recognizing human TLR9, and lysed on ice in RIPA buffer (50 mM Tris-HCl, pH 7.4, 150 mM NaCl, 1% Nonidet P-40, 0.25% Na-deoxycholate, 1 mM EDTA, 1.4 mM Na 3 VO 4 and protease inhibitors). Proteins were immunoprecipitated using anti-human TLR9 (Santa Cruz Biotechnology). Western blot analyses were performed using rabbit anti-human TLR9 (Cell Signaling), rabbit anti-human MYD88, rabbit anti-human TRIF (Alexis), rabbit anti-TRAF3 or rabbit anti-TRAF6 (Cell Signaling Technology). Allergic bronchopulmonary aspergillosis The induction and evaluation of the Th2-driven hypersensitivity response to Aspergillus antigens in the mouse lung has previously been described in detail [26] . Briefly, C57BL/6 or genetically deficient mice were sensitized by the concomitant intraperitoneal (100 μg) and subcutaneous (100 μg) administration of A. fumigatus culture filtrate extract followed 1 week later by the intranasal instillation of 20 μg of the extract. After an additional 7 days, bronchial colonization of A. fumigatus was induced by resting conidia administered intratracheally (1 × 10 7 ), and the animals were evaluated 1 week later for parameters of allergic airway inflammation. Treatments included CpG-ODN administered intraperitoneally (CpG-ODN 1826; 30 μg per mouse twice, on the same days as the first and second administration of A. fumigatus culture filtrate extract). Analysis of respiratory allergy phenotype was as described [35] . Statistical analysis Student’s t -test was used to analyse the results of in vitro studies in which data are mean values (±s.d.). In the in vivo skin test assay, statistical analysis was performed using two-tailed paired t -test by comparing the mean weight of experimental footpads with that of control, saline-injected counterparts [26] . Data are mean values (±s.d.) of three experiments with at least six mice per group per experiment, as computed by power analysis so to yield a power of at least 80% with an α level of 0.05. How to cite this article: Volpi, C. et al. High doses of CpG oligodeoxynucleotides stimulate a tolerogenic TLR9–TRIF pathway. Nat. Commun. 4:1852 doi: 10.1038/ncomms2874 (2013).